Enabling complex nanoscale pattern customization using directed self-assembly Block copolymer directed self-assembly is an attractive method to fabricate highly uniform nanoscale features for various technological applications, but the dense periodicity of block copolymer features limits the complexity of the resulting patterns and their potential utility. Therefore, customizability of nanoscale patterns has been a long-standing goal for using directed self-assembly in device fabrication. Here we show that a hybrid organic/inorganic chemical pattern serves as a guiding pattern for self-assembly as well as a self-aligned mask for pattern customization through cotransfer of aligned block copolymer features and an inorganic prepattern. As informed by a phenomenological model, deliberate process engineering is implemented to maintain global alignment of block copolymer features over arbitrarily shaped, ‘masking’ features incorporated into the chemical patterns. These hybrid chemical patterns with embedded customization information enable deterministic, complex two-dimensional nanoscale pattern customization through directed self-assembly. Through microphase separation, block copolymers (BCPs) can self-assemble into highly uniform, chemically distinct, periodic domains with dimensions and periods at scales of 3–200 nm [1] , [2] that are attractive for nanofabrication. The directed self-assembly (DSA) of BCP thin films using chemical [3] , [4] , [5] , [6] , [7] , [8] or topographical [9] , [10] , [11] , [12] , [13] , [14] , [15] , [16] templates to impose long-range order and registration on the BCP domains has garnered increased interest in recent years as a means to enhance lithographic resolution by multiplying the feature density [5] , [6] , [7] , [8] , [13] , [14] , [15] and rectifying pattern non-uniformity or imperfections [5] , [6] , [17] , [18] of lithographically defined templates. Selective removal or alteration of one block then creates a mask that may be combined with other manufacturing techniques to fabricate devices such as patterned magnetic recording media [19] , silicon nanowire transistors [20] or FinFETs [21] . Successful DSA typically requires commensurability between the spatial frequency of template features and the BCP domain periodicity, which confines its use in lithographic resolution enhancement to the creation of simple, high symmetry, periodic patterns; the limited complexity of such patterns may preclude many envisioned applications. For instance, unidirectional integrated circuit layouts based on a fixed line period [22] may be amenable to the use of DSA-fabricated grating patterns, but such designs still require patterning semi-periodic, isolated and discontinuous features in potentially complicated arrangements on the same layer. This necessitates customization of DSA patterns at very high resolution. This may be accomplished by trimming out lines or portions of lines through additional lithography and etch steps before or after DSA. However, the maximum error tolerance (three times standard deviation, 3σ) for the lithographic overlay alignment required to customize a 28 nm period self-assembled grating pattern is 3 nm [23] . This implies a vanishingly narrow tolerance for overlay misalignment between the DSA and trim patterns as BCP domain sizes useful for patterning approach the sub-10 nm scale. An alternative, self-aligned strategy for generating complex patterns is to form them directly through DSA, avoiding the scaling limits associated with lithographic overlay. This strategy has been demonstrated previously using one-to-one [4] , [24] or two-to-one [25] chemical pattern templates. Complex self-assembled patterns may also be created using sparse topographical templates of post arrays with locally modified spacings, shapes or orientations to adjust the preferred commensurability conditions controlling lateral alignment of BCP domains [14] , [15] , which can be designed using configurable square post lattice template tiles [26] . Even so, the range of possible customizations is restricted, and achieving high target pattern yields is challenging. Here we outline a strategy for precise and complex customizable pattern formation using DSA of BCPs through chemical epitaxy based on two key elements. The first is the use of a hybrid organic/inorganic chemical pattern template including an inorganic ‘prepattern’ with selective affinity for one of the blocks. The affinity allows it to align the BCP, whereas orthogonal etch resistance with respect to at least one of the blocks enables it to serve as a complementary, self-aligned hard mask for further pattern transfer. The second key element is the inclusion in the prepattern of additional non-guiding ‘masking features’ in the inorganic prepattern layer. The thermodynamic drive to minimize free energy enables the BCP to filter out some degree of non-guiding information while preserving global alignment, and so these masking features add a true two-dimensional component to the self-aligned customization afforded by the inorganic prepattern. The composite mask made up of the inorganic prepattern and self-aligned BCP features enable a myriad set of possible customizations. One-dimensional self-aligned customization We demonstrate the basic customization strategy using poly(styrene-block-methyl methacrylate) (PS- b -PMMA) that forms lamellae with a natural period ( L 0 ) of ~25 nm. Additional experimental details may be found in the Methods. The process flow for simple one-dimensional customization is illustrated schematically with corresponding scanning electron microscope (SEM) images in Fig. 1a–h . First, a sparse prepattern is created consisting of thin hydrogen silsesquioxane (HSQ) ‘guiding lines’ patterned by electron beam lithography ( Fig. 1a,b ), where the line-to-line distances are integer multiples ( n ) of the BCP natural period. Underneath the HSQ prepattern is a stack consisting of (from top to bottom) a cross-linked organic layer that enables lamellae to orient perpendicularly to the substrate surface, an inorganic hard mask layer and an organic transfer layer. The HSQ prepattern and the adjacent regions of the exposed cross-linked organic layer together make up the hybrid chemical pattern. A PS- b -PMMA thin film is then cast over the prepattern by spin coating and is thermally annealed for DSA, where the preferential affinity between PMMA and HSQ aligns the lamellae domains in registration with the guiding lines [6] . An oxygen reactive ion etch (RIE) is used to selectively remove the PMMA domains and to break through the orientation control layer, generating a self-assembled mask that is inherently self-aligned with the HSQ prepattern ( Fig. 1c,d ). Together, the HSQ prepattern and the self-aligned mask that are composed of the remaining PS domains make up a single composite mask for further pattern transfer. The seamless nature of this composite mask is afforded by the low placement error between directed BCP domains and the guiding prepattern, which can reach 3σ values of <1 nm [27] . Next, carbon tetrafluoride (CF 4 ) and oxygen RIE steps are used to transfer the composite mask pattern into the underlying inorganic hard mask layer and organic transfer layer ( Fig. 1e,f ). This process thus creates trenches in the organic transfer layer aligned with PMMA domains that were not located over an HSQ prepattern line. Customized line-space patterns are then created through pattern tone inversion using spin-on-dielectric materials ( Fig. 1g,h ). The one-to-one correspondence between the placement of guiding lines in the prepattern and the placement of single-line gaps in the customized line-space pattern shows that the semi-periodic gratings may be readily fabricated by using semi-periodic prepatterns, as demonstrated here. Furthermore, fragmented DSA-generated gratings ( Fig. 1j ) may also be fabricated simply by using fragmented prepatterns ( Fig. 1i ). 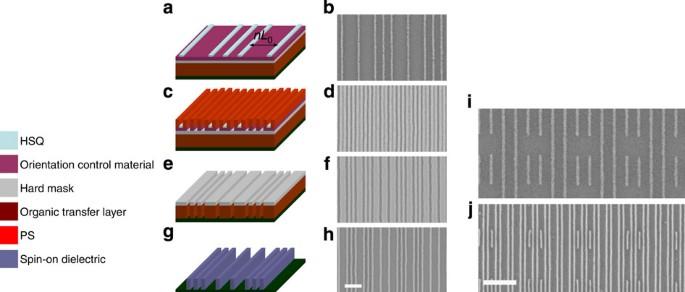Figure 1: Self-aligned, one-dimensional customization. Schematic (a,c,e,g) and SEM images (b,d,f,h) of the fabrication process flow: (a,b) HSQ prepattern. (c,d) DSA and O2RIE to remove PMMA domains. The remaining PS domains and HSQ prepattern form a composite mask for following pattern transfer. (e,f) Pattern transfer of the composite mask into the organic transfer layer using CF4and O2RIEs. (g,h) Pattern tone inversion. (i) SEM image of a fragmented HSQ prepattern and (j) a SEM image of the resulting fragmented DSA-generated grating. Scale bars are 100 nm (b,d,f,h) and 200 nm (i,j). Figure 1: Self-aligned, one-dimensional customization. Schematic ( a , c , e , g ) and SEM images ( b , d , f , h ) of the fabrication process flow: ( a , b ) HSQ prepattern. ( c , d ) DSA and O 2 RIE to remove PMMA domains. The remaining PS domains and HSQ prepattern form a composite mask for following pattern transfer. ( e , f ) Pattern transfer of the composite mask into the organic transfer layer using CF 4 and O 2 RIEs. ( g , h ) Pattern tone inversion. ( i ) SEM image of a fragmented HSQ prepattern and ( j ) a SEM image of the resulting fragmented DSA-generated grating. Scale bars are 100 nm ( b , d , f , h ) and 200 nm ( i , j ). Full size image Challenges in two-dimensional self-aligned customization Although the use of one-dimensional inorganic guiding lines enables customization along the direction of the aligned lamellae period, such guiding features have only limited application for customization in other directions. For true two-dimensional customization, we therefore incorporate a new concept—the addition of non-guiding features into the prepattern. Because these added ‘masking features’ are part of the prepattern, they are also part of the composite mask, including the guiding lines and PS domains that are self-aligned to the guiding lines only. 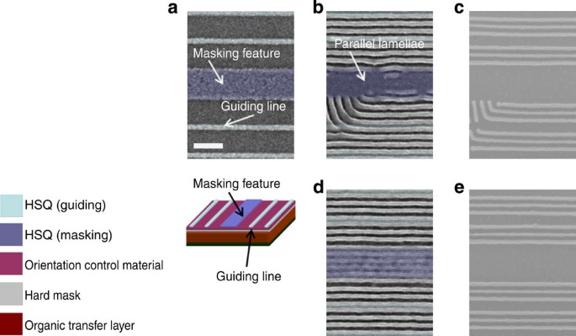Figure 2: Two-dimensional customization using masking features. SEM images of an exemplary prepattern and resulting DSA with pattern transfer and tone inversion under two different conditions. (a) Plan view (upper) and schematic cross-section (lower) of a prepattern including an elongated masking feature. (b) PS-b-PMMA DSA results in the area of that masking feature with parallel lamellae (dark regions), exhibiting poor fidelity with the masking feature dimensions and adjacent misaligned perpendicular lamellae. (c) Pattern transfer and tone inversion after DSA featuring defects similar to those in (b). (d) DSA over the same masking feature with excellent rectification and (e) subsequent pattern transfer and tone inversion. All SEM images are at the same magnification. Dark blue and light blue false colour overlay in (a,b,d) indicate the positions of the masking feature and guiding lines, respectively. Scale bar=100 nm. Figure 2a shows a prepattern consisting of a central elongated HSQ masking feature amidst a guiding line grating designed for frequency quadrupling. The large relative area of the central HSQ masking feature is expected to promote the orientation of lamellae parallel to the substrate to minimize non-preferential interfacial interactions [28] . This local control of lamellae orientation with respect to the chemically patterned substrate has been explored previously as a means to discretize pattern regions or create isolated pattern geometries using one-to-one organic chemical patterns [24] . However, when combined with feature density multiplication, it is challenging to generate reliable and well-defined customizations based on the imperfect orientation control of lamellae using entirely organic chemical patterns [25] . Similar results are observed using these organic/inorganic hybrid chemical patterns. After DSA at 250 °C for 5 min, using a PS- b -PMMA lamellae film 1.2 L 0 thick over the prepattern in Fig. 2a , the dimensions of the nominally parallel lamellae exhibit poor fidelity with respect to dimensions of the prepattern, as shown in Fig. 2b . Moreover, the transition between parallel and perpendicular lamellar regions can cause defects such as misaligned perpendicularly oriented lamellae also shown in Fig. 2b . An advantage to using hybrid chemical patterns is that defects and pattern roughness generated by this perpendicular-to-parallel lamellae transition do not negatively impact pattern transfer using hybrid chemical patterns if they are contained within the area above the masking feature. However, pattern transfer and tone inversion for similarly defective DSA over the same type of masking feature shown in Fig. 2c demonstrate that defects extending beyond the masking feature area propagate into the final pattern. Figure 2: Two-dimensional customization using masking features. SEM images of an exemplary prepattern and resulting DSA with pattern transfer and tone inversion under two different conditions. ( a ) Plan view (upper) and schematic cross-section (lower) of a prepattern including an elongated masking feature. ( b ) PS- b -PMMA DSA results in the area of that masking feature with parallel lamellae (dark regions), exhibiting poor fidelity with the masking feature dimensions and adjacent misaligned perpendicular lamellae. ( c ) Pattern transfer and tone inversion after DSA featuring defects similar to those in ( b ). ( d ) DSA over the same masking feature with excellent rectification and ( e ) subsequent pattern transfer and tone inversion. All SEM images are at the same magnification. Dark blue and light blue false colour overlay in ( a , b , d ) indicate the positions of the masking feature and guiding lines, respectively. Scale bar=100 nm. Full size image Ideally such imperfections can be rectified by ensuring that the masking features are covered by line-space patterns aligned globally by the guiding lines. More simply, DSA is used to form a uniform grating, which is globally aligned by the guiding lines and customized during pattern transfer by the guiding lines and masking features. Although nominally parallel lamellae emerge above large masking features initially during DSA, we have observed that these parallel lamellae regions shrink in area and even disappear as DSA rectification continues, leading to the aforementioned globally aligned grating. An example is illustrated in Fig. 2d , which shows the result of DSA performed at an elevated temperature (265 °C, 5 min, film thickness H =1.2 L 0 ) to accelerate BCP ordering [29] , with excellent rectification above the masking feature, and which generates well-defined customizations on pattern transfer and tone inversion ( Fig. 2e ). Acknowledging the likely presence of an HSQ-wetting layer and possible complex non-bulk morphologies [30] directly above the masking feature, it is clear that these BCP morphologies have negligible impact to pattern transfer outside the masking feature area for complete DSA rectification when using hybrid organic/inorganic chemical patterns. Two-dimensional customization design aspects To enable the design of patterns encompassing a wide range of two-dimensional customizations by DSA using hybrid chemical patterns, it is essential to establish the restrictions on masking feature geometry and the process factors governing rectification. To elucidate the impact of masking feature size, we investigated the isothermal DSA response at 250 °C as a function of annealing time using prepatterns consisting of circular masking features embedded within arrays of guiding lines with a period of 3 L 0 . As an example, Fig. 3a shows a SEM image of a prepattern with an embedded circular masking feature of radius ( R 0 ) 6.6 L 0 along with the response of a thick BCP film ( H ≈1.6 L 0 ) applied onto the prepattern after different annealing times. Initially the parallel lamellae regions shrink at a slow rate. After 10 min, the regions shrink rapidly. Half of the parallel lamellae regions formed over this size-masking feature had disappeared within 15 min, and the remaining instances (shown in the SEM image) from our data set had reduced in size, considerably. Within 20 min, most parallel lamellae regions corresponding to masking features with R 0 =6.6 L 0 had been rectified. 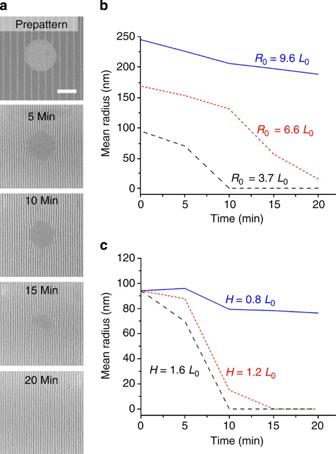Figure 3: Influence of masking feature size on rectification. (a) Time series SEM images of parallel grains above a circular masking feature withR0=6.6L0. (b) Parallel grain mean radii versus annealing time for three differently-sized circular masking features atH≈1.6L0. Lines indicate mean values, starting from the mean masking feature radius. (c) Circular parallel lamellae grain mean radii versus annealing time using three BCP film thicknesses (H) forR0=3.7L0. The graphical depiction of all data pertaining to (b) through (c) is located inSupplementary Figure 1. Scale bar=200 nm. Figure 3: Influence of masking feature size on rectification. ( a ) Time series SEM images of parallel grains above a circular masking feature with R 0 =6.6 L 0 . ( b ) Parallel grain mean radii versus annealing time for three differently-sized circular masking features at H ≈1.6 L 0 . Lines indicate mean values, starting from the mean masking feature radius. ( c ) Circular parallel lamellae grain mean radii versus annealing time using three BCP film thicknesses ( H ) for R 0 =3.7 L 0 . The graphical depiction of all data pertaining to ( b ) through ( c ) is located in Supplementary Figure 1 . Scale bar=200 nm. Full size image The dependence of the time required for rectification on masking feature size for a film thickness of H ≈1.6 L 0 is evident in the DSA response using different sized masking features. This is depicted graphically in Fig. 3b , which shows the radii of parallel lamellae regions that formed initially above masking features of different R 0 as a function of annealing time. For R 0 =6.6 L 0 , complete rectification occurs in ~15 to 20 min. For R 0 =3.7 L 0 , complete rectification occurs in <10 min, whereas for R 0 =9.6 L 0 , the parallel lamellae region continue to shrink but never disappear within a 20 min annealing time. Importantly, as time progresses, the rate of change of the parallel lamellae region radii sometimes increases, particularly for smaller radii, indicating an inverse relationship between rectification speed and radii of the parallel lamellae regions. Film thickness is also a key factor for DSA rectification. Its influence is revealed in a comparison of parallel lamellae region radii above R 0 =3.7 L 0 masking features as a function of annealing time for three different film thicknesses ( H ≈1.6, 1.2 and 0.8 L 0 ), shown in Fig. 3c . The parallel lamellae regions appear to shrink more slowly for H ≈1.2 L 0 than for H ≈1.6 L 0 , though complete rectification occurs in most cases within a 10 min annealing time. As BCP film thickness is reduced further to H ≈0.8 L 0 , the parallel lamellae region is rectified even more slowly and complete rectification never occurs. This behaviour is a consequence of the preferential affinity between PMMA and HSQ that favours the formation of parallel lamellae to minimize interfacial energy. This energetic penalty to rectification becomes more prominent as the interfacial free energy becomes a larger fraction of the total system free energy in a thinner film. Such rectification behaviour can be understood in the context of BCP grain coarsening, where a lamellae grain with an initial parallel orientation over the masking feature at the beginning of thermal annealing shrinks over time to reduce the free energy imparted by the presence of a grain boundary between parallel lamellae over the masking features and surrounding globally aligned perpendicular lamellae. In analogy to abnormal grain growth in thin films of polycrystalline semiconductors [31] , the shrink rate ( v ) for circular parallel-lamellae grains of radius r can be modelled as ( Supplementary Discussion for derivation): Shrinkage of the parallel grain is driven by the reduction of grain boundary energy, γ GB / r , where γ GB is the grain boundary interfacial tension. It is impeded by the net free energy penalty per unit volume, arising as lamellae transition from a parallel to a substantially perpendicular orientation over preferentially wetted masking features (Δ f ( H )), which reflects both HSQ-PMMA preferential affinity and the effects of BCP thin-film confinement. The 1/ r dependence in the grain boundary energy term can explain our observation that the radii of smaller grains shrink faster than those of larger ones. In addition, the magnitude of Δ f diminishes with increasing BCP film thickness ( H ) as the BCP film becomes more bulk-like and the HSQ-BCP interface assumes less of a role in determining the total system free energy. The shapes of masking features are also key elements, determining restrictions in prepattern design for this customization scheme. To investigate their effects on rectification, we used single masking features designed with different aspect ratios but approximately the same areas (35,000±7,000 nm 2 ; ~56L 0 2 ) embedded in the centers of gratings with 3 L 0 period guiding lines. 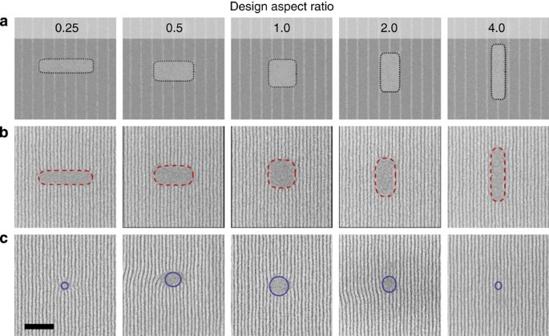Figure 4: Influence of masking feature shape on rectification. (a–c) SEM images of HSQ masking features with the same approximate areas but different aspect ratios (a) and the results of DSA at film thicknessesH≈0.8L0(b) andH≈1.0L0(c). The overlying red dashed lines in (b) and blue solid lines in (c) represent parallel grain contours calculated as described in theSupplementary Methodsafter annealing for high and low relative Δf/γGBvalues, respectively, according to the model described in the main text and theSupplementary Discussion. The initial contours used for calculation are represented by the dotted black lines overlying the masking features in (a). Scale bar =200 nm. Figure 4a–c shows SEM images of masking features with aspect ratios ranging from 0.25 to 4.0 ( Fig. 4a ) along with the DSA response after 5 min thermal annealing (250 °C) at H ≈0.8 L 0 ( Fig. 4b ) and H ≈1.0 L 0 ( Fig. 4c ), where it is apparent that the thicker film exhibits more dramatic rectification, especially at extreme aspect ratios. For even thicker films ( H ≥1.2 L 0 ), the initial parallel lamellae grains were completely rectified for all aspect ratios. The observed dependence of the speed of rectification on grain aspect ratio can also be explained in the shrinking grain model by the relative magnitude of energy penalty with respect to the grain boundary interfacial tension (Δ f/γ GB ), where r represents the local radius of curvature of parallel grains in the substrate plane. This is shown by model calculations of parallel lamellae grain contours after BCP annealing ( Supplementary Methods ), overlying the SEM images of DSA patterns in Fig. 4b,c (initial contours used for calculations are depicted by the dotted black lines overly the masking features in Fig. 4a ). Within the model, rectification proceeds at similarly slow speeds for all aspect ratios in a thinner film with a higher magnitude of Δ f/γ GB (0.045nm −1 ; Fig. 4b , red dashed line), whereas in a thicker film with a lower relative magnitude of Δ f/γ GB (0.015nm −1 ; Fig. 4c , solid blue line), rectification proceeds noticeably faster for rectangles (both low and high aspect ratios) than squares as a result of the higher curvature on the short sides for rectangles. However, for negligible Δ f (Δ f/γ GB ≈0), the areas of all lamellae grains shrink at approximately the same, faster rate regardless of aspect ratio ( Supplementary Methods and Supplementary Figs 2 and 3 ). As Δ f/γ GB diminishes with increasing film thickness, the masking feature shapes used in prepattern designs exert minimal impact on the rectification process when DSA conditions are engineered to minimize Δ f/γ GB , as is the case for thick BCP films. Therefore, with the proper choice of BCP film thickness, there are very few restrictions on the shapes of the masking features used to customize DSA arrays. Figure 4: Influence of masking feature shape on rectification. ( a – c ) SEM images of HSQ masking features with the same approximate areas but different aspect ratios ( a ) and the results of DSA at film thicknesses H ≈0.8 L 0 ( b ) and H ≈1.0 L 0 ( c ). The overlying red dashed lines in ( b ) and blue solid lines in ( c ) represent parallel grain contours calculated as described in the Supplementary Methods after annealing for high and low relative Δ f/γ GB values, respectively, according to the model described in the main text and the Supplementary Discussion . The initial contours used for calculation are represented by the dotted black lines overlying the masking features in ( a ). Scale bar =200 nm. Full size image Enabling complex two-dimensional customization So far, we have demonstrated that simple pattern customizations are made possible by establishing process conditions in which BCP grain boundary energy minimization can overcome the energy penalty imposed by the preferential chemical affinity of the prepattern to realize global BCP alignment over masking features in the hybrid chemical pattern. Now, we demonstrate the applicability of this technique to more complex customizations. An example of an elaborate customization is shown in Fig. 5a , which is an SEM image of a prepattern containing nine 240 nm (~10 L 0 ) wide and 520 nm (~21 L 0 ) long masking features outlining the letters ‘IBM’ ( Fig. 5e ). The prepatterns investigated include 3 L 0 period guiding lines, maintaining commensurability in the area surrounding each masking feature; under ideal rectification eight PMMA (and nine PS) domains line up across the masking feature during DSA. 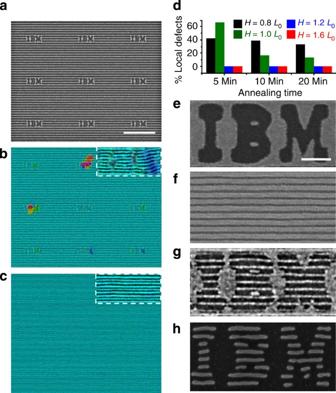Figure 5: Complex bidirectional customization. (a–cande–h) SEM images of the prepattern and resulting DSA patterns. (b) and (c) are overlaid with their corresponding false colour-orientation maps. (a) HSQ prepattern incorporating a masking feature outlining the letters ‘IBM’. (b) DSA pattern after PMMA removal forH≈1L0after 5 min. thermal annealing at 265 °C. Inset: zoomed-in view of the area with ‘IBM’. (c) DSA pattern after PMMA removal forH≈1.6L0after 5 min. thermal annealing at 265 °C. Inset: zoomed-in view of the area with ‘IBM’. (d) Plot of the fraction of the ‘IBM’s featuring defects local to the IBM region for the DSA patterns atH≈0.8, 1.0, 1.2 and 1.6L0against the corresponding thermal annealing time period. (e) Zoomed-in view of the area with ‘IBM’ in (a). (f) DSA pattern after PMMA removal forH≈1.2L0after 5min. thermal annealing at 265°C over the ‘IBM’ logo based on the prepatterns in (a). (g) Facsimile of the IBM logo in a grating generated through DSA atH≈1.2L0based on the prepattern in (a). (h) Tone-inverted IBM logo generated through DSA. Scale bars are 1 μm (a–c) and 100 nm (e–h). Figure 5b,c show the results of DSA using H ≈1.0 L 0 and H ≈1.6 L 0 BCP films, respectively, at an elevated temperature (265 °C) to increase ordering speed. In Fig. 5b,c , the BCP pattern is superimposed with its false colour lamellae orientation map [32] , [33] , [34] , providing a spatial map of lamellae alignment (or misalignment). Previously, lamellae line-space patterns have been observed to display a tendency to orient orthogonally to borders between regions of strong chemical contrast [30] , [35] , [36] ; this tendency imposes an initial ‘local alignment’ on lamellae within or nearby the letters. With decreasing rectilinearity of each letter’s borders with respect to the global alignment direction from left to right, the local and global alignment directions increasingly conflict, presenting greater difficulty for defect free rectification across the masking feature. In thinner films ( H ≈1.0 L 0 , Fig. 5b ), some lamellae on the masking features remain horizontal to the substrate and misaligned or defective grating patterns are introduced as a result of the conflicting local alignment within the masking feature areas. In contrast, a globally aligned line-space pattern is formed over masking features in thicker films ( H ≈1.6 L 0 ) at 5 min of annealing time ( Fig. 5c ). To quantitatively analyze the effect of BCP film thickness and DSA annealing time, with the use of prepatterns depicted in Fig. 5a , we classify the images with defects as seen in the Fig. 5b inset as ‘defective’ with a value of 1 and those as in the Fig. 5c inset as ‘not-defective’ with a value of 0. A plot of the fraction of defects over time for ~100 test prepatterns as a function of annealing time and the BCP film thickness is shown in Fig. 5d . The local defectivity for H ≈0.8 L 0 remains unchanged with increasing time at ~40% defectivity, whereas although the local defectivity for H ≈1.0 L 0 decreases with increasing thermal annealing time, it only diminishes to ~15% within 20 min. On the other hand, thicker films ( H ≈1.2 L 0 , 1.6 L 0 ) show no local defects after only 5 min annealing. Figure 5: Complex bidirectional customization. ( a – c and e – h ) SEM images of the prepattern and resulting DSA patterns. ( b ) and ( c ) are overlaid with their corresponding false colour-orientation maps. ( a ) HSQ prepattern incorporating a masking feature outlining the letters ‘IBM’. ( b ) DSA pattern after PMMA removal for H≈ 1 L 0 after 5 min. thermal annealing at 265 °C. Inset: zoomed-in view of the area with ‘IBM’. ( c ) DSA pattern after PMMA removal for H≈ 1.6 L 0 after 5 min. thermal annealing at 265 °C. Inset: zoomed-in view of the area with ‘IBM’. ( d ) Plot of the fraction of the ‘IBM’s featuring defects local to the IBM region for the DSA patterns at H ≈0.8, 1.0, 1.2 and 1.6 L 0 against the corresponding thermal annealing time period. ( e ) Zoomed-in view of the area with ‘IBM’ in ( a ). ( f ) DSA pattern after PMMA removal for H ≈1.2 L 0 after 5min. thermal annealing at 265°C over the ‘IBM’ logo based on the prepatterns in ( a ). ( g ) Facsimile of the IBM logo in a grating generated through DSA at H ≈1.2 L 0 based on the prepattern in ( a ). ( h ) Tone-inverted IBM logo generated through DSA. Scale bars are 1 μm ( a – c ) and 100 nm ( e – h ). Full size image Figure 5e–h emphasizes the process for fabricating high resolution, complex two-dimensional customized patterns through DSA. Figure 5e shows a zoomed-in view of an area with ‘IBM’ in Fig. 5a , whereas Fig. 5f shows a DSA pattern generated after PMMA removal for conditions conducive to rectification ( H ≈1.2 L 0 , annealed at 265 °C for 5 min) over the ‘IBM’ logo. A carefully timed etch for the sample in Fig. 5f ( Fig. 5g ) reveals the BCP domains superimposed with the underlying HSQ masking features and shows superior BCP healing with no distortions as compared with Fig. 5b . Pattern transfer and tone inversion then results in a facsimile of the IBM logo with feature sizes approaching 10 nm, such as the example shown in Fig. 5h . High-resolution, deterministically customized two-dimensional patterns can be generated though DSA in a straightforward way when customization features and DSA conditions are designed such that grain boundary energy minimization is the dominant driving force for forming globally aligned BCP arrays over hybrid chemical patterns. In summary, we have shown that hybrid organic/inorganic chemical patterns including guiding and non-guiding (masking) elements can be used to direct the self-assembly of BCPs for fabricating arbitrarily customizable arrays. The self-assembled features are self-aligned to guiding prepattern features and rectify non-guiding prepattern features by a process of grain boundary energy minimization. Based on this mechanism, customization of DSA arrays can be done simply using straightforward process engineering and chemical pattern design rules. The strategy presented here is general, and we anticipate that its use may be extended to other BCPs with non-lamellar morphologies, and even to other nanomaterials that self-assemble in ensembles to create a variety of non-canonical patterns. Initial applications of this strategy are likely to be most relevant to the patterning needs of the semiconductor industry, but the large variety of customizable, semi-periodic nanopatterns available through this technique may amplify the usefulness of DSA in burgeoning technological applications like the fabrication of plasmonic or photonic devices [37] , [38] . Materials and procedures Lamellae forming PS- b -PMMA (M n =22 kg mol −1 –22 kg mol −1 ; M w /M n =1.09) was purchased from Polymer Source and used as received. The natural period of the lamellae ( L 0 ) was determined by Fourier transform analysis of SEM images of fingerprint patterns occurring naturally in areas of the sample away from prepattern. Its mean value of 25.5 nm varied by <3% (2σ) across all samples investigated. The pattern tone inversion material was a spin-on-dielectric (NFC IRM 007-6) obtained from JSR Micro. The material stack for pattern transfer consisted of (bottom to top) an organic transfer layer, an inorganic hard mask and an orientation control layer used to orient the PS-PMMA lamellae perpendicularly with the substrate. Each layer was deposited by spin coating. The organic transfer layer (HM 8500) was obtained from JSR Micro and the hard mask was a silicon-containing anti-reflective coating (SHB-A940) obtained from Shin-Etsu Chemical. The orientation control material was poly(styrene-r-epoxydicyclopentadiene methacrylate), synthesized by traditional free-radical polymerization in methyl ethyl ketone, using 2,2'-azobis(2-methylpropionitrile) initiator. Using a styrene:epoxydicyclopentadiene methacrylate feed ratio=75:25, the polymer had M n =4,800 kg mol −1 , M w /M n =1.50. The styrene:epoxydicyclopentadiene methacrylate molar ratio is ~74:26 by inverse-gated 13C NMR. The epoxydicyclopentadiene monomer used in this work was originally obtained as a research sample from Elf Atochem. It was redistilled before use. The monomer can be prepared using the general route described by Allen et al . [39] The intermediate dicyclopentadienyl methacrylate is commercially available from Sartomer, Inc. (product ID: CD535). For casting on a substrate, the orientation control material was combined in solution with N -(trifluoromethylsulfonoxy)phthalimide thermal acid generator (10 wt% relative to polymer) in propylene glycol methyl ether acetate. Si wafers with a ~1 μm thick SiO 2 layer and the pattern stack described above were spin-coated with a 6 nm thick orientation control layer that was cross-linked by baking at 220 °C for 5 min in air. HSQ resist was spin-coated on top of this orientation control layer. Subsequent patterning by electron beam lithography was used to create the prepatterns 3–5 nm in height, with guiding lines ~15 nm (~0.6 L 0 ) wide. The height of HSQ guiding lines (~0.16 L 0 ) adds a degree of topography to the chemical pattern that may complicate normal chemical epitaxy-based DSA. However, we observed that the BCP responds in much the same way to the chemical pattern used here as another BCP did in our previous work [6] in which the guiding line height was noticeably less (~2 nm, ~0.07 L 0 ).The guiding line period was preset as an integer multiple of L 0 to maintain commensurability with the BCP natural period; in the majority of cases guiding lines with a period of 3 L 0 were used. Before DSA, the HSQ patterns were cured by baking for 15 min in air at 215 °C to tune their surface energy [40] for optimal BCP ordering. PS-PMMA films ~20 to 40 nm thick were then spin-coated from 2% (w/w) in propylene glycol methyl ether acetate solutions, and film thicknesses were measured from SEM cross-sectional images. For DSA, samples were thermally annealed at different temperatures for various times. The samples depicted in Fig. 2b,c in the main text were annealed at 250 °C in air for 5 min. The samples from which SEM images were acquired in Figs 1 and 2d,e , were annealed at 265 °C under N 2 purge for 5 min. The samples from which SEM images were acquired in Fig. 5 were annealed at 265 °C under N 2 purge for various times. All other samples were annealed at 250 °C under N 2 purge for various times. PS and PMMA were etched to various extents by oxygen RIE(~2:1 PMMA:PS etch rate ratio) for various times. Pattern transfer was accomplished using CF 4 and oxygen RIEs. For pattern tone inversion, the tone inversion material was spun onto the pattern in the organic transfer layer. The tone inversion material and hard mask were etched back using a CF 4 RIE to reveal the organic transfer layer. The organic transfer layer was then removed using an oxygen RIE. The density of the ‘IBM’ masking features investigated was chosen to obtain reliable statistics while allowing independent rectification above each masking feature. Higher densities of masking features may also affect rectification and is the topic of further study beyond the scope of this work, but we found that a 67% increase in the density of the ‘IBM’ masking features resulted in no increase in local defectivity after DSA (265 °C, 20 min.) with H≈1.6 L 0 . Variability in the pattern transfer and pattern tone inversion steps independent of the DSA process were observed. High yield of the tone-inverted DSA structures can be achieved by proper co-optimization of the material stack, etch and fill processes, using tooling typically available for high-volume semiconductor manufacturing, as exemplified by Tsai et al . [21] , [41] Image analysis SEM images were obtained using a Leo 1550 field emission SEM, and image analysis was performed using ImageJ. Smoothing and background suppression were accomplished simultaneously using a band pass filter. Image contrast was enhanced by normalizing the range of pixel intensities to the maximum intensity range, and images were binarized by thresholding at 50% of the maximum range. For prepattern images, the threshold was inverted. Masking features and parallel lamellae grains were isolated by repeated erosion operations followed by the same number of repeated dilation operations. For rectangular masking features, aspect ratios were obtained from the areas ( A ) and the second moment of areas ( I xx or I yy ). Actual measured aspect ratios differed from the design aspect ratios by <15%. For circular masking features, radii ( r ) were obtained from the relation . How to cite this article: Doerk, G. S. et al . Enabling Complex Nanoscale Pattern Customization Using Directed Self-Assembly. Nat. Commun. 5:5805 doi: 10.1038/ncomms6805 (2014).